Quantifying thiol–gold interactions towards the efficient strength control The strength of the thiol–gold interactions provides the basis to fabricate robust self-assembled monolayers for diverse applications. Investigation on the stability of thiol–gold interactions has thus become a hot topic. Here we use atomic force microscopy to quantify the stability of individual thiol–gold contacts formed both by isolated single thiols and in self-assembled monolayers on gold surface. Our results show that the oxidized gold surface can enhance greatly the stability of gold–thiol contacts. In addition, the shift of binding modes from a coordinate bond to a covalent bond with the change in environmental pH and interaction time has been observed experimentally. Furthermore, isolated thiol–gold contact is found to be more stable than that in self-assembled monolayers. Our findings revealed mechanisms to control the strength of thiol–gold contacts and will help guide the design of thiol–gold contacts for a variety of practical applications. Self-assembled monolayers (SAMs) of thiols on gold surfaces are one of the most popular model systems for the study of the self-assembly of organic molecules on metal surfaces. SAMs that are based on thiol–gold chemistry have been widely employed in the fields of chemistry, physics, molecular biology, pharmaceutical engineering and materials science [1] , [2] , [3] . Considerable interests in such systems have increased, owing to their versatile applications, including the fabrication of nanopatterning [4] , [5] , molecular-scale devices [6] , [7] , optical materials [8] , [9] , formulation of biosurfaces [10] and support for cell culture [2] , [11] . The strength of the gold–sulphur (Au–S) interaction formed between thiols and gold surfaces provides the basis to fabricate robust SAMs for diverse applications. The study on the nature of Au–S interaction and the stability of SAMs formed on gold surfaces under various conditions, such as different surface properties of gold, solution pH and types of solvents, is thus important. One of the effective ways for such study is to break the individual Au–S contact by external force. Given the limited availability of detection methods, such experiments are challenging. The advent of several single-molecule manipulation techniques, including optical tweezers, magnetic tweezers, biomembrane force probe and atomic force microscopy (AFM)-based single-molecule force spectroscopy (SMFS), offers new and powerful tools to investigate the intra- or intermolecular interactions of both natural (biological) and synthetic macromolecules [12] , [13] , [14] , [15] , [16] . These interactions are unbinding forces that originated from specific interactions in biological systems (that is, the unfolding of proteins, melting of DNA strands, antigen–antibody interactions, ligand–receptor interactions and protein–nucleic acid interactions), entropic elasticity, basic supramolecular interactions (that is, hydrogen bonds, coordinated bonds, π – π interactions, hydrophobic interactions and so on) and even the strength of a single covalent bond [13] , [17] , [18] , [19] , [20] , [21] , [22] , [23] , [24] , [25] , [26] , [27] , [28] . The investigations of molecular interactions in complicated systems, such as on live bacterial surfaces, in intact virus particle, and in condensed polymer materials, have also been performed successfully via AFM-based SMFS [21] , [22] , [29] . For thiol–gold interactions, numerous investigations focusing on the exploration of the rupture mechanism of Au–S interaction have been carried out in the past few years by using both experimental and theoretical methods. Gaub et al. [24] pioneered in conducting SMFS experiments to detect the strength of a single covalent bond around Au–S binding sites. They determined a rupture force of 1.4±0.3 nN in their experiments. However, they did not answer unambiguously the origin of the measured rupture force (that is, the rupture of the Au–S bond or the extraction of the anchored gold atoms from substrates). Ab initio molecular dynamics simulations [30] , [31] in the framework of ‘virtual AFM experiments’ demonstrate that pulling a thiol attached to the gold surface could result in the breakage of a Au–Au bond with rupture force of ~\n1.2 nN. Mechanically controlled break-junction experiments [32] , [33] that are slightly different from the AFM-based force experiments have demonstrated that the breaking of the molecular junctions takes place at Au–Au bonds near the molecule–electrode contact and produces a similar rupture force of 1.5 nN. However, an AFM-based force experiment conducted by Skulason et al. [25] showed a small force value of 0.1 nN, which was also demonstrated to be the abstraction of thiolate–complexed gold atoms from the tip surface. Recently, Venkataraman et al. [34] measured the breaking force in thiol junctions and showed a rupture force of ~\n1.0 nN. These results show that the forces required to break the Au–Au bonds obtained in their respective experiments are substantially different from each other, although the underlying rupture mechanism is thought to be identical in these different experiments. A careful comparison of these studies shows that the experimental conditions, gold surface properties and sample preparation conditions (solvent and pH) are actually different. This observation implies that significant variations in rupture forces between these measurements may originate from different experimental conditions. This finding also suggests that the strength of a single Au–Au bond around Au–S binding sites can be influenced by external factors. Investigating the factors that affect the strength of thiol–gold contact is necessary to clarify these controversial results. This approach can also facilitate a deep and direct understanding of the rupture mechanisms and dynamic processes of a single bond formed between thiol and gold surfaces, as well as the rational design of stable novel nanomaterials and nanodevices based on Au–S-specific interaction. However, to the best of our knowledge, detailed information on the fundamental factors affecting the strength of single bonds formed between Au and S atoms of thiol for both isolated single molecules and individual molecules in SAMs, especially at the single molecular level, remains unavailable. In this paper, AFM-based SMFS is employed to study the effects of experimental conditions on the strength of single bonds at the thiol–gold interface formed by isolated thiols or in SAMs. Our results show that thiolate-bound gold atoms could be extracted from the gold surface with the retraction of the AFM tip, leading to the breakage of Au–Au bonds near the Au–S binding sites for both isolated thiols and SAMs. For isolated thiols, the strength of single bonds formed between thiols and Au surfaces is strongly affected by the properties of the gold surface, the solution pH and the interacting time. We also observe a shifting of the bond from coordinate to covalent bond upon increasing the environmental pH and the interaction time. However, the strength of individual Au–Au bonds around Au–S binding sites for SAMs is affected only by the properties of the gold surface and the reaction time. Our results also show a large difference in the rupture forces of Au–Au covalent bonds obtained from isolated thiols and individual thiols in SAM. The significance of our findings is discussed. Effect of surface properties on thiol–gold contacts Proper cleaning of the gold surface is necessary to obtain high-quality thiol–gold-based SAM. For this purpose, rational methods for preparing highly reproducible gold surfaces, including the oxidative [35] , [36] , [37] , [38] and reductive [36] , [37] pretreatments, have been proposed. Briefly, gold substrates could be oxidized to a positive charge state via conventional methods, such as ultraviolet/ozone, oxygen plasma, electrochemical oxidation and piranha solution oxidation. The freshly prepared oxidized gold surfaces can be chemically reduced to zero state (metallic gold) after they were immersed in ethanol. Given that these pretreatment methods could produce different states (valence) of gold surfaces, correlating the gold properties with the stability of thiol–gold contact is necessary. To the best of our knowledge, no such study at the single molecule level is currently available. In this section, the effects of the properties of gold surfaces on the strength of single thiol–gold contacts at pH 8.0 are discussed. As described above, oxidized and reduced gold surfaces were prepared by employing piranha solution and ethanol, respectively, to study this effect. In accordance with the phenomena reported in literature, the oxidized gold substrates were hydrophilic, whereas the reduced gold substrates were hydrophobic [39] , [40] . X-ray photoelectron spectroscopy (XPS) was used to precisely determine the oxidization states of the freshly prepared gold surfaces. As seen in Fig. 1 , the Au 4f 7/2 bands with binding energies of 84.85 and 83.95 eV correspond to oxidized and reduced gold surfaces, respectively, which indicate that the ethanol treatment changed the gold surface from the oxidized to the reduced state. The narrow scans in the Au 4 f region of oxidized gold surface shifted to higher binding energy compared with the reduced surface [36] , [41] , [42] , indicating a remarkable energy difference between each doublet. 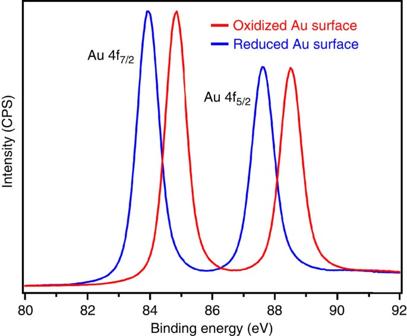Figure 1: XPS evidence for the oxidization and reduction of gold surfaces. The spectra represent the two sets of doublet (4f7/2and 4f5/2) of Au 4f core-level spectra of oxidized (red line) and reduced (blue line) gold surfaces. Figure 1: XPS evidence for the oxidization and reduction of gold surfaces. The spectra represent the two sets of doublet (4f 7/2 and 4f 5/2 ) of Au 4f core-level spectra of oxidized (red line) and reduced (blue line) gold surfaces. Full size image α -Thiol- ω -carboxy-terminated poly (ethylene glycol) (HS-PEG-COOH) was attached to the amino-group-modified AFM tip via the amide bond, leaving the thiol ends exposed for attachment to the gold surface. During the contact of thiol-labelled AFM tip with the gold substrate (oxidized or reduced), a molecular bridge formed between the AFM tip and the gold substrate via the thiol–gold chemistry ( Fig. 2a ). During the separation of the AFM tip with the gold surface, the weakest part of the bridge structure broke, resulting in a rupture event. The resulting rupture force was measured ( Fig. 3 ). Statistical analysis on the rupture forces was performed. 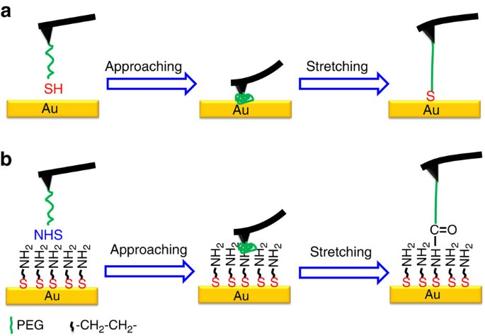Figure 2: Illustration of AFM-based SMFS study of the gold–sulphur interactions. (a) Illustration of the formation and breakage of isolated thiol–gold contactin situ. (b) Illustration of the detection of thiol–gold interactions in amino-terminated, self-assembled monolayers. Figure 2: Illustration of AFM-based SMFS study of the gold–sulphur interactions. ( a ) Illustration of the formation and breakage of isolated thiol–gold contact in situ . ( b ) Illustration of the detection of thiol–gold interactions in amino-terminated, self-assembled monolayers. 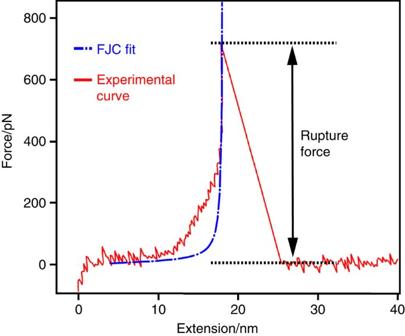Figure 3: Typical force–extension curve with the freely jointed chain (FJC) fit. The rupture forces obtained on such single molecule stretching curves were employed to construct the force histograms. The deviation between the experimental curve and FJC fit is due to the PEG linker66. Full size image Figure 3: Typical force–extension curve with the freely jointed chain (FJC) fit. The rupture forces obtained on such single molecule stretching curves were employed to construct the force histograms. The deviation between the experimental curve and FJC fit is due to the PEG linker [66] . 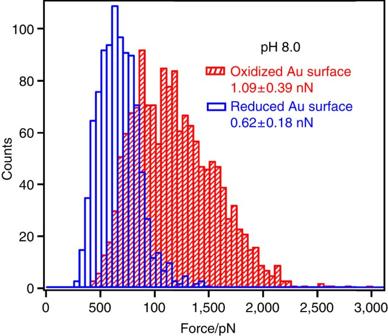Figure 4: Effect of surface properties on the strength of thiol–gold contacts at pH 8.0. Histograms of the rupture forces obtained by unbinding the isolated thiol from the oxidized (red) (n=1,510,nis number of events) and reduced (blue) (n=970) gold surfaces at pH 8.0. Full size image Figure 4 shows the histograms of rupture forces obtained on oxidized and reduced gold surfaces at pH 8.0, respectively. For the oxidized gold surface, the most probable rupture force is 1.09±0.39 nN. For the reduced gold surface, the force histogram indicates a most probable rupture force of 0.62±0.18 nN. Previous studies [5] , [27] , [30] , [31] , [32] , [34] , [43] , [44] strongly indicated that the breakage takes place at the Au–Au bond around the Au–S binding sites, which was the weakest among the covalent bonds (that is, Si–O, Si–C, C–N, C–C, C-O, Au–S and Au–Au) in the linkage, leaving one or more gold atoms at the terminal of the tethered linker. Control experiments, in which the thiol-terminated PEG was replaced with sulphur-free methoxyl-terminated PEG, were performed to confirm that the rupture force obtained above originated from the interaction between the sulphydryl group and gold surfaces. The histograms of the resulted rupture forces obtained from the interaction between PEG-OCH 3 linker and gold surfaces gave force peaks of 43 pN at pH 7.4 and 34 pN at pH 8.0, respectively (see Supplementary Fig. 1 ). Figure 4: Effect of surface properties on the strength of thiol–gold contacts at pH 8.0. Histograms of the rupture forces obtained by unbinding the isolated thiol from the oxidized (red) ( n =1,510, n is number of events) and reduced (blue) ( n =970) gold surfaces at pH 8.0. Full size image Another control experiment on sulphydryl-terminated silicon surface ( Fig. 5 ) indicates that the gold atoms have been extracted from the gold surface and became attached to the AFM tip during the pulling experiment (see Fig. 5a and Supplementary Fig. 2 ). Based on these facts, we deem that the obtained rupture force shown in Fig. 4 can be ascribed to the cleavage of single Au–Au bonds. 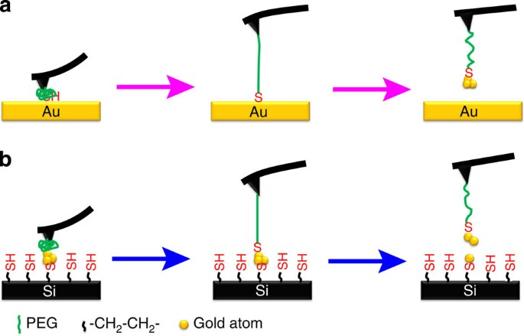Figure 5: Illustration of AFM-based SMFS study of the breakage of isolated Au–Au bonds. (a) Illustration of the abstraction of gold atoms from the gold surfaces. (b) Same AFM tip employed inawas brought to interact with the sulphydryl-terminated silicon surfaces. Figure 5: Illustration of AFM-based SMFS study of the breakage of isolated Au–Au bonds. ( a ) Illustration of the abstraction of gold atoms from the gold surfaces. ( b ) Same AFM tip employed in a was brought to interact with the sulphydryl-terminated silicon surfaces. Full size image Although the rupture of the same bonds on stretching is very likely to be in both cases, the most probable rupture force obtained on oxidized gold surfaces is larger than that on the reduced surfaces. As proposed by Ron et al. [37] , thiols may directly react with the oxidative gold surface to form Au–S bonds via the oxidation–reduction reaction involving the reduction of the gold oxide and the direct adsorption of thiols onto the reduced gold surface. The formed species on both the oxidized and reduced gold surfaces are gold (I) thiolates. Different variation in the degree of valence may have distinct effects on the precise rearrangement behaviour of the gold atoms beneath the surface, which in turn could result in the variation of the strength of the Au–Au bond. Recently, ab initio investigations [45] on the formation of alkanethiol on gold surfaces suggested the existence of a noticeable perturbation of the position of the gold atoms around the Au–S binding sites, which affect the electronic structures of the neighbouring gold atoms. The difference of the unbinding force in our current system may thus come from the different rearrangement of the surrounding gold atoms on oxidized and reduced gold surfaces during the binding process. Effect of pH on the strength of single thiol–gold contacts The adsorption of thiol onto gold surface starts with physisorption, during which the H atom favourably remains on the S atom, followed by a chemisorption including the breaking of S–H bond and the formation of a Au–S bond as a result of the deprotonation of thiols and formation of thiyl radicals [45] , [46] , [47] , [48] , [49] , [50] , [51] . The existence of the dissociated hydrogen could affect the pH value of the microenvironment around the Au–S binding sites. Thus, the environmental pH also affects the formation of the Au–S bond, because an acidic environment inhibits the dissociation of S–H bonds, whereas an alkaline environment favours this dissociation. To the best of our knowledge, no detailed/direct information exists on the effect of environmental pH on dynamic processes for the formation of Au–S covalent bonds. AFM-based SMFS method was employed to quantify the effect of pH on the mechanical strength of an isolated thiol–gold contact. 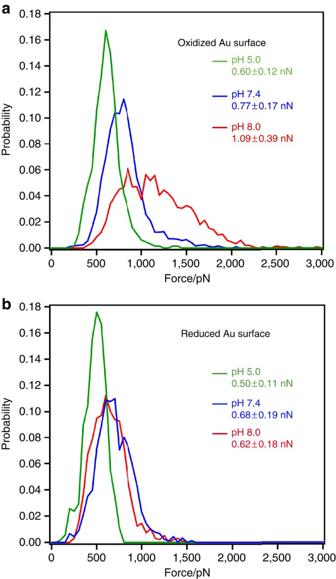Figure 6: pH effects on the strength of thiol–gold contacts. Histograms of the forces required to rupture single bonds formed between isolated thiols and (a) oxidized and (b) reduced Au surfaces at pH 5.0 (green line), 7.4 (blue line) and 8.0 (red line), respectively. Figure 6 shows the distributions of rupture forces of thiol–gold contacts obtained on oxidized ( Fig. 6a ) and reduced ( Fig. 6b ) gold surfaces in aqueous solutions at different pH values, respectively. From the data, we can see that the bonds formed between isolated individual thiols and oxidized gold surfaces break with a most probable unbinding force of ~\n0.60, 0.77 and 1.09 nN at pH 5.0, 7.4 and 8.0, respectively. The most probable corresponding rupture forces obtained on reduced gold surfaces are ~\n0.50, 0.68 and 0.62 nN, respectively. The most probable rupture force obtained on oxidized gold surfaces increases with increasing pH value. The rupture forces obtained on reduced gold surfaces show a minimum force value at pH 5.0 and similar force values at pH 7.4 and 8.0, respectively. Figure 6: pH effects on the strength of thiol–gold contacts. Histograms of the forces required to rupture single bonds formed between isolated thiols and ( a ) oxidized and ( b ) reduced Au surfaces at pH 5.0 (green line), 7.4 (blue line) and 8.0 (red line), respectively. Full size image During the formation of a Au–S covalent bond, multiple bonding scenarios exist depending on the location of the H atom, which could lead to drastic changes in the rupture force [44] , [52] , and a possibility of forming weaker coordinate bonds between the protonated SH groups and gold surfaces [53] . Recently, a comprehensive investigation on the elongation process of molecular junctions formed by octanedithiol molecule and Au electrodes indicated that the bonds that are easiest to break are the coordinated Au-linker contacts (~\n0.6 nN), which are smaller than the covalent thiolate–gold junctions (from ~\n1.5 to ~\n2.2 nN) [52] . These findings indicate that the fraction of the intact –SH group could have great influence on the rupture force obtained in SMFS experiments. Considering the reaction mechanisms between thiols and gold surfaces, a higher proportion of intact –SH groups, which could form Au–SH coordination bonds, can most probably exist at lower pH values. On the contrary, more –SH groups deprotonated and the percentage of Au–S covalent bonds increased significantly at higher pH conditions, leading to a larger rupture force. As a result, the increase in pH value would shift the bond type of thiol–gold contact from a coordinate bond to a covalent bond. To further prove our hypothesis, both XPS and Raman spectroscopy have been used to study thiol–gold interactions and the main findings are in good agreement with our SMFS results (see Supplementary Figs 3 and 4 ). The higher rupture force observed on oxidized gold surface may be ascribed to the fact that the presence of gold oxide (for example, the –OH groups on the surface) promotes the conversion of the protonated SH group to water in the reaction, whereas the released proton remains in the form of hydrogen ions for the reduced gold surface. Effect of interaction time on thiol–gold contacts As discussed above, the coordinate bond could actually form between the –SH group and gold surface in the initial stage, followed by the dissociation of S–H bond that results in a thiyl radical, which would finally form a gold–thiolate covalent bond at the gold–sulfur interface [45] , [46] , [47] , [48] , [49] , [50] , [51] , [54] , [55] , [56] , [57] , [58] . These findings indicate that the formation of Au–S covalent bonds needs a certain time to complete. Experimental evidence [58] also suggests that the loss of hydrogen can be prevented to some extent as long as no reaction occurs for hydrogen removal, which provides a way to control the bonding strength between thiols and gold. By changing the waiting/reaction time during the contact of the thiol group and gold surfaces, we have investigated the effects of interaction time on the strength of thiol–gold interaction at the single molecule level. 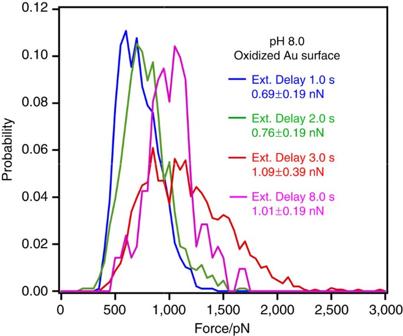Figure 7: Interaction time dependence of the strength of thiol–gold contacts. Histograms of the forces required to rupture single bonds formed between thiol and oxidized gold surfaces at pH 8.0 with increase of surface waiting time from 1.0 s to 2.0, 3.0 and 8.0 s. Figure 7 shows histograms of the rupture forces obtained between thiols and gold surfaces at pH 8.0 with different interaction times. The most probable rupture forces of 0.69 nN at 1.0 s, 0.76 nN at 2.0 s, 1.09 nN at 3.0 s and 1.01 nN at 8.0 s have been observed. The rupture forces increased with the increase of interaction time from 1.0 to 3.0 s. This finding indicates that an apparent shifting of bond types from coordinate to covalent with the increase in the interaction time might have occurred. Figure 7: Interaction time dependence of the strength of thiol–gold contacts. Histograms of the forces required to rupture single bonds formed between thiol and oxidized gold surfaces at pH 8.0 with increase of surface waiting time from 1.0 s to 2.0, 3.0 and 8.0 s. Full size image The rupture force obtained at the interaction time of 8.0 s is also similar to that obtained at 3.0 s, which indicates that after a reaction time of ≥3.0 s, the majority of the thiol–gold contact will form a covalent bond at pH 8.0. The quantitative information obtained on the stability of isolated thiol–gold contacts by using AFM-based SMFS is useful for sample systems where the strength of individual thiol–gold contact plays important roles, such as the picking up (or immobilization) and manipulation of thiol-labelled polyethylene oxide chain (or polyprotein) [22] , [59] , [60] . An in situ waiting time of ≥3.0 s for the formation of covalent S–Au bond is necessary to stabilize the thiol–gold chemistry-based molecular linkages. Strength of individual thiol–gold contacts in SAMs From the discussion above, we know that experimental conditions can significantly affect the stability of the isolated thiol–gold contacts. How much will these conditions affect the stability of the thiol–gold contacts in SAMs? To answer this question, SAMs of amino-terminated thiol have been prepared on oxidized and reduced gold surfaces, respectively; environmental conditions, such as surface properties, pH and reaction time, on its stability were also studied by using the SMFS method ( Fig. 2b ). It needs to be pointed out that we focus on the quantitative comparison of the stability of the thiol–gold contact in isolated state and in SAMs in this study. To realize this, we need to minimize the effect of neighbouring/adjacent molecules in SAMs on the apparent thiol–gold interactions (or the apparent rupture forces obtained by AFM). Thus, we have chosen cysteamine, which contain short carbon chain, for the preparation of SAMs, since thiol molecule with long alkane chain will further stabilize the SAMs [2] , [60] . A survey on the published papers shows that the commonly used reaction time for the preparation of SAMs of thiols on gold surfaces ranged from a few minutes to days. In accordance with frequently used reaction conditions published in literature, SAMs employed in our experiments were prepared by immersing oxidized or reduced Au substrates in 100 mM of cysteamine PBS (pH 7.4) solution for 0.5, 5.0 and 24 h, respectively. Subsequently, the mechanical stability of SAMs was studied by using AFM-based SMFS at pH 8.0. 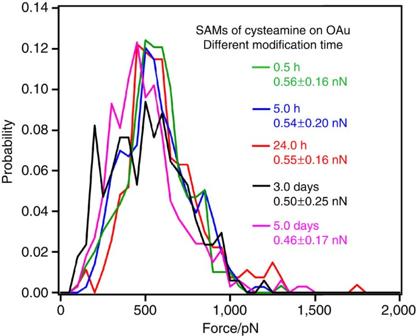Figure 8: Effect of reaction time on stability of thiol–gold contacts in SAMs. Histograms of the rupture forces obtained from the SAMs, which were produced by immersing oxidized Au substrates in 100 mM of cysteamine solutions for 0.5 (green line), 5.0 (blue line), 24.0 h (red line), 3 days (black line) and 5 days (pink line). SMFS experiments were carried out at pH 8.0. Figure 8 shows the most probable rupture forces of 0.56 nN for 0.5 h, 0.54 nN for 5.0 h and 0.57 nN for 24.0 h for SAMs formed on oxidized gold surface. No significant variation of the rupture forces was observed, suggesting similar mechanical stability for them. A further prolonged reaction time, for example, 5 days, can even weaken the thiol–gold interactions so that the rupture force can reach ~\n0.46 nN, which is close to that obtained on reduced gold surface, as shown in Supplementary Fig. 5 . This result indicates that from the stability point of view, 0.5 h is enough for the formation of SAMs, and very long reaction time is not helpful. The information is useful for the immobilization of sensitive thiol-containing proteins (or other biological samples) on gold substrate [18] . Figure 8: Effect of reaction time on stability of thiol–gold contacts in SAMs. Histograms of the rupture forces obtained from the SAMs, which were produced by immersing oxidized Au substrates in 100 mM of cysteamine solutions for 0.5 (green line), 5.0 (blue line), 24.0 h (red line), 3 days (black line) and 5 days (pink line). SMFS experiments were carried out at pH 8.0. Full size image By using a similar experimental strategy, we also investigated pH effects on the stability of the SAMs formed on oxidized and reduced gold surface, respectively. The most probable rupture forces for the breaking of individual molecules in SAMs on oxidized Au surfaces are 0.55 nN at pH 5.0, 0.53 nN at pH 7.4, and 0.57 nN at pH 8.0, respectively (see Supplementary Fig. 6a ). The force profile corresponding to the rupturing force of individual molecules in SAMs on reduced gold surfaces indicates the most probable rupture forces of 0.49 nN at pH 5.0, 0.48 nN at pH 7.4, and 0.46 nN at pH 8.0 (see Supplementary Fig. 6b ). Our results reveal that the rupture force obtained on an oxidized gold surface is larger than that obtained on a reduced gold surface at the same pH value. Another important phenomenon is that the most probable bond rupture force does not change with the change of the solution pH on respective gold surfaces. Considering the fact that the SAMs were formed by 5-h reaction at pH 7.4, the cleavage of S–H bond and the formation of Au–S covalent bond should be completed. As a result, the solution pH will not affect the binding (between the thiol and gold) process any more. Control experiments, in which the same AFM tip that has been used to break the thiol–gold contacts in SAMs ( Fig. 2b and Supplementary Fig. 7 ), were used to perform the force measurement on sulphydryl-terminated silicon surface again to prove our hypothesis. The result shows that the Au–Au bond has been broken, and gold atoms were attached to the AFM tip during the force measurement on SAMs (see Supplementary Fig. 7 , top row). In addition, it is interesting to note that the rupture force obtained in the control experiment (~\n1.2 nN) (Step II) is bigger than that obtained in Step I (~\n0.57 nN) (see Supplementary Fig. 7 ). This phenomenon may indicate that the arranging modes of Au atoms on the gold substrate are different from that attached to the AFM tip (more like gold nanocluster). Furthermore, it has been recognized that Au(111)/SAM interface can contain a layer of Au adatoms that are covalently bonded with the neighbouring thiol(ate) molecules, that is, the first atomic layer above a metallic Au(0) surface contains a layer of Au(I) and S. This bonding network is covalent (–(S–Au) n –) [1] , [61] . Hence, when the AFM tip is contacted to a thiol(ate) that is a part of the SAM layer, a possible scenario where a complex molecular wire was peeled off from the gold substrate and get attached to the AFM tip would happen, as shown in the bottom row of Supplementary Fig. 7a . The breakage of such kind of molecular wire in Step II can happen either at the Au–Au or the Au–S sites, depending on the binding mode between thiol group (on the silicon surface) and the molecular wire of gold (see Supplementary Fig. 7b,c ). As a result, the histogram may shift towards higher force values and get broadened. Our results also indicate that after the formation of SAMs, environmental pH will not affect the stability of the SAMs. However, during the formation of SAMs, the solution pH can affect the efficiency for the conversion of thiol–gold contacts from non-covalent (that is, coordinate) to covalent bonds (see Supplementary Figs 3 and 4 ). These findings are useful for the design of gold nanoparticle and thiol–gold chemistry-based drug (or gene) delivery systems. 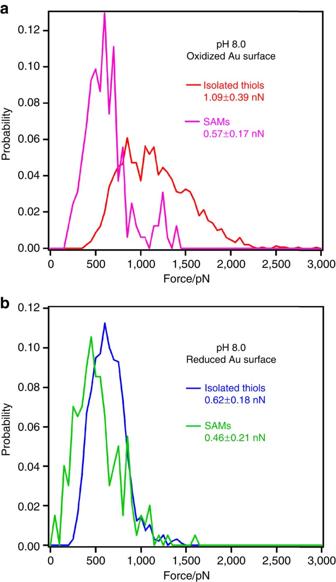Figure 9: Comparison of the strength of isolated thiol–gold contacts and that in SAMs. Histograms of rupture forces of the single thiol–gold contact formed by isolated molecules and in SAMs on (a) oxidized and (b) reduced gold surfaces at pH 8.0, respectively. Comparison of isolated thiol–gold contacts and that in SAMs Figure 9 shows the direct comparison of the mechanical strength of single thiol–gold contacts formed by isolated single thiols and in SAMs on oxidized ( Fig. 9a ) and reduced ( Fig. 9b ) surfaces at pH 8.0, respectively. Interestingly, our results show that the rupture forces of isolated single molecules immobilized on both oxidized and reduced gold substrates are larger than that obtained on SAMs formed on respective substrates. For oxidized gold surfaces ( Fig. 9a ), the most probable rupture force obtained from an isolated molecule (~\n1.09 nN) is significantly larger than that obtained in SAMs (~\n0.57 nN). For reduced gold surfaces ( Fig. 9b ), the most probable rupture force obtained from an isolated molecule (~\n0.62 nN) is also larger than that obtained in SAMs (~\n0.46 nN). Figure 9: Comparison of the strength of isolated thiol–gold contacts and that in SAMs. Histograms of rupture forces of the single thiol–gold contact formed by isolated molecules and in SAMs on ( a ) oxidized and ( b ) reduced gold surfaces at pH 8.0, respectively. Full size image The formation of a Au–S covalent bond is a complicated process, involving the dissociation of the S–H bond and followed by the formation of the Au–S covalent bond [45] , [46] , [47] , [48] , [49] , [50] , [51] . The dissociated hydrogen atoms could either adsorb on gold surfaces or release from the surface in the form of H 2 . Ensemble experiments also indicated that the loss of hydrogen could undergo a very slow process [56] , [58] , even as long as several minutes, which is longer than the interaction time (3.0 s) between isolated thiols and gold surfaces in our SMFS experiments for isolated thiols. The released H located on the gold surface could lead to drastic changes in rupture forces [45] , [52] . These facts have caused the dependence of the unbinding force on pH and waiting time (within the time scale of 3.0 s) for isolated thiol–gold contacts. However, the SAMs adopted in our experiments were prepared by immersing the freshly prepared oxidized or reduced gold substrates into 100 mM of cysteamine aqueous or alcoholic solutions for 5 h at room temperature, respectively. The dissociated H from the SH group would have detached from the gold surfaces and have no effect on the rupture force of Au–Au bond in our experiments. The large difference of rupture forces of the thiol–gold contacts formed by isolated and self-assembled thiols may be ascribed to the following reasons: (1) the large amount of cysteamine (100 mM) can act as a reduction reagent, and the originally oxidized gold surface has been reduced during the formation of SAMs (see Supplementary Fig. 8 ). As discussed above, the reduced gold surface can weaken the Au–Au bond; (2) the formation of SAMs on gold surfaces may weaken the interactions between gold atoms in the top and lower layers because earlier scanning tunnelling microscopy studies have shown the mobility of Au thiolates within the SAMs of alkanethiols [62] , [63] . We have quantified the effects of experimental conditions, such as surface properties, solution pH/composition and reaction time, on the strength of chemical bonds formed between isolated thiols and gold surfaces or those in SAMs by using AFM-based SMFS. Our results unambiguously demonstrate that an oxidized gold surface can significantly enhance the stability of thiol–gold contacts in both isolated and self-assembled systems. However, for the later case, if the reaction time during the formation of SAMs on oxidized gold is too long (for example, longer than 5 days), the enhancement of stability will decrease greatly (see Fig. 8 ). This may indicate that the final molecular structures of the Au/SAM interface on oxidized and reduced gold are similar, as the XPS spectra of these two system are very similar (see Supplementary Fig. 8 ). When ethanol is adopted as the solvent during the preparation of SAMs on oxidized gold surface, the strength of thiol–gold contacts can be weakened because of the reduction effect of ethanol on gold. The formation of covalent thiol–gold contacts shows pH dependence: at lower pH, coordinate bonds dominate in the contacts; at higher pH, the bond type becomes covalent. Our results also show that the in situ formation of Au–S covalent bond requires a minimal interaction time of around 3.0 s. This observation means that to obtain a stable molecular bridge in between a gold-coated AFM tip and the substrate via the thiol–gold chemistry, a contact time of 3.0 s is necessary. Although the direct contact of thiol-modified AFM tip with gold substrate can speed up the reaction between the thiol and gold (as compared with the reaction in free solution) due to the shorter mass transport time, normally higher indentation force (>200 pN) will not speed up the reaction further, and indentation force that is too high may even destroy the thiol group or the PEG linker. Considering the fact that the time for mass transport in our AFM experiment is nearly zero, the 3.0 s interaction time necessary for strong interaction is the formation of covalent Au–S bonds [25] , [55] . However, the reaction time for the formation of SAMs can be different. Depending on the type of thiol molecules (for example, with long or short alkyl chain), the concentration as well as the cleanness of the gold surface, the formation time for a ‘full monolayer’ can vary from seconds to minutes, up to hours and days [2] , [55] , [64] . The weakened strength of the thiol–gold contact in SAMs compared with that of isolated thiols can be ascribed to both the reduction effect of the thiols and the further weakening effect of the self-assembled thiols on the Au–Au interactions. Our findings on the stability of thiol–gold contacts are useful for practical applications. For example, to stabilize the anchor of single thiol-labelled molecules, we can use an oxidized gold surface and perform the reaction in aqueous (rather than in ethanolic) solution at higher pH with appropriate reaction time (for example, ~\n3.0 s for isolated thiol–gold contacts, while less than 1 day for SAMs). For the single-molecule pulling experiment, in which a thiol-labelled molecule needs to be attached to the gold substrate and the strength of the thiol–gold contact is crucial to the experiment [18] , [60] , the molecule of interest needs to be immobilized onto the gold surface under a more dilute solution; the utilization of small thiol molecules as a ‘dilute agent’ is also avoided to co-assemble the target molecule [13] . Chemicals and reagents HS-PEG-COOH (Mw=3,400 Da, PDI=1.4) and ω -carboxy-terminated poly (ethylene glycol) methyl ether (Mw=20,000 Da, PDI=1.05) were purchased from Polymer Source Inc. α , ω -dicarboxyl-terminated poly (ethylene glycol) (HOOC-PEG-COOH, Mw=3,500 Da, PDI=1.03) was purchased from JenKem Technology Co. 3-Aminopropyldimethylmethoxysilane was obtained from Fluorochem (UK). (3-Mercaptopropyl)trimethoxysilane, N-hydroxy-succinimide (NHS), 1-(3-dimethylaminopropyl)-3-ethylcarbodiimide hydrochloride (EDC) and cysteamine were purchased from Sigma-Aldrich. The PBS solution (pH 7.4) was prepared by dissolving one PBS tablet (Sigma) in 200 ml of deionized water and filtered. All other chemical reagents were of analytical reagent grade and were used as received without further purification. High-purity deionized water (dH 2 O>18 MΩ cm) purified with a Millipore System was adopted to prepare all aqueous solutions in this work. Silanization of AFM tips Silicon nitride AFM tips (Veeco Instruments, now Bruker Nano, Santa Barbara, CA; MSCT) with different functionalizations were employed for the SMFS experiments. Before modification, the AFM tips were treated with piranha solution (H 2 SO 4 (98%)/H 2 O 2 (30%)=7:3 in volume), followed by thorough rinsing with high-purity deionized water, and then drying in an oven at 115 °C for 90 min to remove any remaining water. ( Caution: Piranha solution that may result in explosion or skin burns is a very hazardous oxidant. This solution must be handled with extreme care. ) The vapour-phase deposition method was introduced to silanize the cleaned AFM tips by suspending them in the atmosphere of the 3-aminopropyldimethylmethoxysilane in a dry nitrogen-purged desiccator for 1 h at 20 °C. After rinsing thrice with methanol, the silanized tips were subsequently placed in a 110 °C oven for 10 min. Thiol derivatization of AFM tips The thiol-terminated tips were prepared by introducing a covalent attachment of thiol-bearing polymer (HS-PEG-COOH) to amino-terminated AFM tips using standard EDC/NHS chemistry. Briefly, the carboxyl ends of the PEG (0.1 mM) were activated by reacting with EDC (6.0 mM) and NHS (10 mM) in PBS at pH 7.4 to introduce succinimide-reactive groups. The activated polymer was incubated with the amino-functionalized tips for 1 h and was then rinsed thrice with PBS (pH 7.4) to remove unanchored molecules. NHS activation of AFM tips HOOC-PEG-COOH was activated by employing EDC/NHS chemistry as described above before use. Afterwards, the amino-silanized tips were incubated with the resulting 4.2 mM α , ω -di(NHS)-PEG in PBS buffer for 30 min. The tips were rinsed thrice with the same buffer to remove unanchored molecules. Preparation of oxidized gold surfaces Gold surfaces (with ~\n50 nm of chromium and 200 nm of gold on glass substrate) were degreased for 5 min in anhydrous ethanol and then placed in freshly prepared piranha solution (H 2 SO 4 (98%)/H 2 O 2 (30%)=7:3 in volume) for at least 10 min. The gold surfaces were rinsed with high-purity deionized water exhaustively and dried with high-purity nitrogen gas. The freshly prepared gold substrates were termed oxidized gold substrates. Preparation of reduced gold surfaces The reduced gold substrates were obtained by immersing the freshly prepared oxidized gold substrates in pure anhydrous ethanol for 2 h at room temperature. Preparation of amino-terminated SAMs Amino-terminated SAMs on oxidized gold surfaces were prepared by immersion of the oxidized gold substrate in 100 mM of cysteamine PBS (7.4) solution for 5 h. The SAMs on reduced gold surfaces were prepared by immersion of the reduced gold sample in 100 mM of ethanolic solution of cysteamine for 5 h. Afterwards, the samples were carefully rinsed with deionized water and dried with high purity nitrogen. Preparation of sulphydryl-terminated silicon substrate Silicon wafers were first treated with freshly prepared piranha solution (H 2 SO 4 (98%)/H 2 O 2 (30%)=7:3 in volume), followed by thorough rinsing with high-purity deionized water, and drying in an oven at 115 °C for 90 min to remove any remaining water. ( Caution: Piranha solution that may result in explosion or skin burns is a very hazardous oxidant. This solution must be handled with extreme care. ) The vapour-phase deposition method was introduced to silanize the cleaned silicon substrates by suspending them in the atmosphere of (3-mercaptopropyl)trimethoxysilane in a dry nitrogen-purged desiccator at 25 °C for 120 min. Subsequently, wafers were rinsed thrice with methanol, followed by drying under a stream of nitrogen gas. AFM-based SMFS Force spectroscopy experiments on both isolated single molecules ( Fig. 2a ) and individual molecules in SAMs ( Fig. 2b ) on gold were carried out on a NanoWizardII BioAFM (JPK Instrument AG, Berlin, Germany) in contact mode. Detailed descriptions on the operation of the AFM-based SMFS have been reported elsewhere [13] , [21] , [22] . Functionalized Si 3 N 4 AFM tips were adopted in this work, and the spring constants of AFM cantilevers were calibrated by the thermal noise method, producing spring constants of 0.02–0.03 N m −1 (ref. 65 ). All measurements were carried out with freshly prepared AFM tips and samples in PBS buffer at room temperature. In each approach–retraction cycle, a modified AFM tip was first brought into contact with the gold surface at a constant indentation force of 200 pN and then held on the gold surface for 3.0 s, unless stated otherwise before retraction. During the separation of the AFM tip from substrate, the formed connective bridge in-between can be stretched and eventually broken, and the rupture force can be recorded. The pulling speed was kept constant at 1.0 μm s −1 for all experiments. Analysis of SMFS data Considering that PEG spacer was employed during the pulling experiment, force-extension curves that show characteristic mechanical properties of a single PEG chain (that is, those that show only a single rupture event, can be fitted by the modified freely jointed chain model below 100 pN and above 300 pN region with a fixed Kuhn length of 7 Å, and with the typical kink at around 300 pN [66] ) were analysed ( Fig. 3 ). Histograms of the rupture forces were fitted by a Gaussian function to obtain the most probable unbinding forces. All data analyses were performed by using custom software written in Igor Pro. (Wavemetrics). X-ray photoelectron spectroscopy XPS spectra were collected by using an electron spectrometer (ESCALAB 250) equipped with monochromatized Al Kα radiation source with pass energy of 30 eV. The binding energies were corrected by referencing the C (1s) 284.6 eV. How to cite this article: Xue, Y. et al. Quantifying thiol–gold interactions towards the efficient strength control. Nat. Commun. 5:4348 doi: 10.1038/ncomms5348 (2014).